Crown ethers in graphene Crown ethers are at their most basic level rings constructed of oxygen atoms linked by two- or three-carbon chains. They have attracted attention for their ability to selectively incorporate various atoms or molecules within the cavity formed by the ring. However, crown ethers are typically highly flexible, frustrating efforts to rigidify them for many uses that demand higher binding affinity and selectivity. Here we present atomic-resolution images of the same basic structures of the original crown ethers embedded in graphene. This arrangement constrains the crown ethers to be rigid and planar. First-principles calculations show that the close similarity of the structures should also extend to their selectivity towards specific metal cations. Crown ethers in graphene offer a simple environment that can be systematically tested and modelled. Thus, we expect that our finding will introduce a new wave of investigations and applications of chemically functionalized graphene. Almost a half century ago, the introduction of crown ethers [1] created a sensation by demonstrating that weakly coordinating ether atoms held together in large molecular rings could selectively bind alkali metal cations. The implications for a new ‘host-guest’ chemistry stirred the imagination of chemists with exciting possibilities of tailoring molecules with cavities whose size, shape and donor properties would allow for the capture of any desired guest species for seemingly boundless applications [2] , [3] , [4] , [5] , [6] , [7] , [8] , [9] , [10] , [11] . Since its discovery as a stable two-dimensional material in 2004 (ref. 12 ), graphene has been widely and actively explored in the hopes of functionalizing this remarkable material [13] , [14] , [15] . Graphene oxide is the most-studied form of functionalized grapheme [16] , [17] . It is believed that graphene oxide to a first approximation consists of defective graphene sheets with oxygen-containing epoxy and hydroxyl groups on the surface and carboxylic, hydroxyl and carbonyl groups at the sheet edges [18] . Controlled chemical [19] or thermal [20] reduction of graphene oxide has also been shown to provide tunability of the electronic [21] , [22] , [23] and optical [24] properties. Hossain et al. [25] have shown that it is possible to produce a chemically homogeneous and reversible form of graphene with epoxy functionalization. However, the structure of the as-prepared graphene oxide and, thus, its corresponding properties are metastable because of continuous desorption of weekly bonded oxygen from graphene even at room temperature [26] . Reduced graphene oxide is largely pristine graphene that contains significant amounts of residual oxygen (~8–10 at. % [19] , [24] ) even after high-temperature annealing (800–1,100 °C) or long time chemical reduction. We have studied the most stable oxygen–carbon complexes. Despite high-resolution electron microscopy studies of the local oxygen–carbon atomic configurations present in graphene oxide [25] , [27] , [28] , it has been NMR, infrared absorption and electron diffraction that so far have provided the best information on the oxygen bonding configurations in graphene oxide [29] , [30] , [31] . One reason for this is that only the most strongly bound configurations can withstand the high-energy electron beam in an electron microscope. The most stable oxygen–carbon groups were thought to be present at the edge of the graphene oxide sheets [18] . However, the only image of oxygen in graphene that we have found in the literature to date is in the work of Zan et al. [27] , where an oxygen atom is imaged incorporated in the graphene lattice after a hole is refilled with migrating absorbed carbon atoms and an oxygen impurity atom. Here using aberration-corrected scanning transmission electron microscopy (STEM) [32] , we obtained direct images of the atomic configurations of what we calculate to be the most stable oxygen atoms incorporated in graphene. Maarouf et al. [33] have recently shown that using first-principles calculations that n-doping of graphene can be achieved by adding K or Na to an O-passivated pore created by removing 12 carbon atoms. Crown ether structures Crown ether molecules are often presented as prototypical host molecules, but in fact this family of compounds has proved limited in binding strength and selectivity. In contrast to the flat two-dimensional drawings of crown ethers typically shown with all of the oxygen atoms lining a central cavity ( Fig. 1a ), the ether dipoles do not actually point directly at the guest ion within the three-dimensional cavity ( Fig. 1b–d ). Consequently, the electrostatic energy realized on binding is much smaller than what is available if the dipoles could converge completely without strain. Another limitation arises from the flexibility of the crown ether rings, which gives rise to an entropic cost in reorganizing the molecule to open its cavity from its natural shape typically lacking a cavity ( Fig. 1e ). The reorganization often introduces significant ring strain, which adds a further energy cost to ion binding [34] . Cram [9] elegantly demonstrated the extremely high binding affinity that can be obtained by rigidifying (that is, ‘preorganizing’) the host molecule. 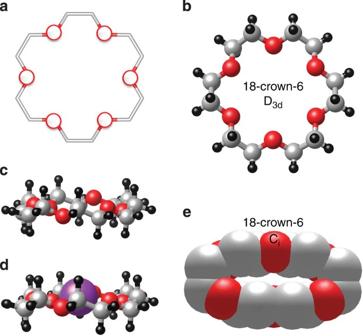Figure 1: Atomic structures of crown molecules with different symmetry (D3dand Ci). (a) Typical two-dimensional representation of 18-crown-6, so-named by Pedersen1. (b) Top view and (c) side view of 18-crown-6 in its crown-shaped D3dsymmetry (H atoms are black and O atoms are red). The C–O–C dipoles imperfectly converge towards the central cavity. (d) Side view of K+ion captured within 18-crown-6 with D3dsymmetry with C–O–C dipoles slightly rotated toward the K+ion but still only at a grazing angle. (e) Top view of 18-crown-6 (van der Waals radii) as crystallized with Cisymmetry, no cavity, and divergent C–O–C dipoles. Figure 1: Atomic structures of crown molecules with different symmetry (D 3d and C i ). ( a ) Typical two-dimensional representation of 18-crown-6, so-named by Pedersen [1] . ( b ) Top view and ( c ) side view of 18-crown-6 in its crown-shaped D 3d symmetry (H atoms are black and O atoms are red). The C–O–C dipoles imperfectly converge towards the central cavity. ( d ) Side view of K + ion captured within 18-crown-6 with D 3d symmetry with C–O–C dipoles slightly rotated toward the K + ion but still only at a grazing angle. ( e ) Top view of 18-crown-6 (van der Waals radii) as crystallized with C i symmetry, no cavity, and divergent C–O–C dipoles. Full size image Experimental structures Medium-angle annular dark-field (ADF) imaging in an aberration-corrected STEM combined with electron energy-loss spectroscopy (EELS) reveals that our graphene oxide samples contain detectable amounts of Si, O and C (see Supplementary Fig. 1 ). Most of the Si and O are found to be located in the thicker amorphous-looking layers on the graphene. Si is also found at edges of the graphene sheets. However, no trace of oxygen at the investigated edges was detected. Oxygen atoms were found in graphene only at the edges of small holes in the graphene lattice. These small holes along with paired five- and seven-atom defects are the most common lattice defects found in the single layers of graphene oxide that we examined. The five- and seven-atom defects (two-dimensional dislocations) appear to be the result of reconstructions of multisite vacancies in graphene layers [32] . 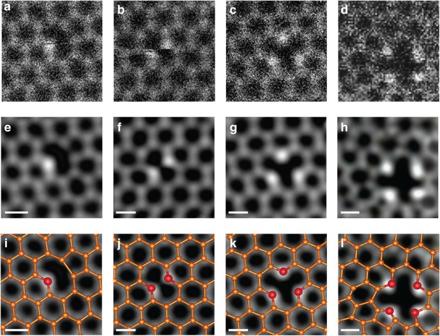Figure 2: Atomic structures of oxygen atoms incorporated in graphene multivacancies. (a–d) Experimental STEM-ADF Z-contrast images of oxygen atoms (one, two, three and four, respectively) in graphene multivacancies. (e–h) Experimental STEM-ADF Z-contrast images of oxygen atoms processed to remove noise and probe-tail effects. (i–l) Calculated structures overlaid on the corresponding ADF images, for the defects shown ina–d, respectively. Scale bar, 0.2 nm. Figure 2a–d shows the ADF images of oxygen atoms incorporated in graphene multivacancies. Figure 2: Atomic structures of oxygen atoms incorporated in graphene multivacancies. ( a – d ) Experimental STEM-ADF Z-contrast images of oxygen atoms (one, two, three and four, respectively) in graphene multivacancies. ( e – h ) Experimental STEM-ADF Z-contrast images of oxygen atoms processed to remove noise and probe-tail effects. ( i – l ) Calculated structures overlaid on the corresponding ADF images, for the defects shown in a – d , respectively. Scale bar, 0.2 nm. Full size image Calculated structures First-principles calculations of the relaxed structures are superimposed on the experimental images Fig. 2i–l . The binding energy of oxygen in these configurations is ~9.0 eV. Under 60 keV electron beam irradiation, the maximum energy transfer to an oxygen atom is about 8.1 eV [35] . This is the reason that we are able to directly observe this stable oxygen configuration in graphene. The oxygen atoms present in graphene oxide as epoxy and hydroxyl groups have lower binding energy (3.75 eV/O and 1.5 eV/OH) and are therefore removed during investigation by electron microscopy. To understand how the observed structures are formed, calculations of multi-atom vacancies in graphene before and after oxygen incorporation were performed. 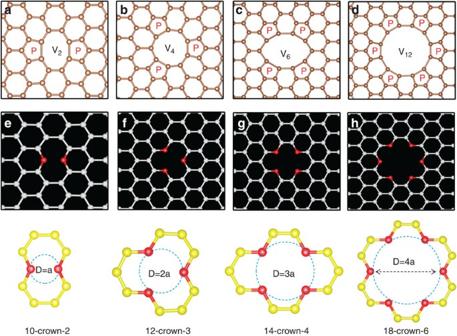Figure 3: Calculated structures of multi-atom vacancies in graphene before and after oxygen incorporation. (a–d) the relaxed atomic models of multivacancies in graphene (double, tetra, hexa and dodeca, respectively). ‘P’ indicates the five-atom rings and Vnindicates the number of vacancies. (e–h) sequence of resulting crown ether structures after oxygen incorporation. Cavity diameter is indicated, in which ‘a’ is the C–C distance (~1.426 Å). Figure 3 shows that the oxygen is incorporated in the pentagonal carbon rings formed in multi-atom vacancies in graphene. The resulting C–O configurations closely resemble simple crown ether molecules as seen in Fig. 3e–h . Figure 3: Calculated structures of multi-atom vacancies in graphene before and after oxygen incorporation. ( a – d ) the relaxed atomic models of multivacancies in graphene (double, tetra, hexa and dodeca, respectively). ‘P’ indicates the five-atom rings and V n indicates the number of vacancies. ( e – h ) sequence of resulting crown ether structures after oxygen incorporation. Cavity diameter is indicated, in which ‘a’ is the C–C distance (~1.426 Å). 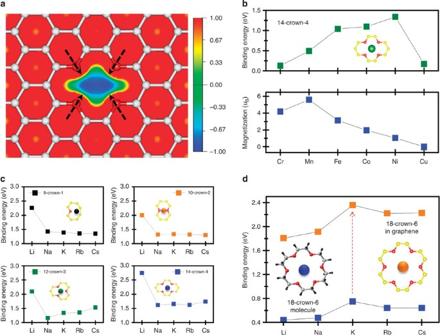Figure 4: Electrostatic potential and selectivity of crown ethers incorporated in graphene. (a) Two-dimensional contour plot of electrostatic potential (normalized by maximum value) of 14-crown-4. (b) Binding energy of various transition metals in the 14-crown-4 structure in graphene (c) Binding energy of alkaline atoms to the 9-crown-1, 10-crown-2, 12-crown-3 and 14-crown-4 structures in graphene. (d) Binding energy of alkaline atoms in the 18-crown-6 structure in graphene exceeds that of free 18-crown-6 molecules by about 1.4 eV. Full size image Figure 4a shows the calculated in-plane electrostatic potential (normalized by maximum value) of 14-crown-4 in graphene. We find that the ether dipoles, specified in black arrows, are all aligned on the level of the sheet, maximizing the binding energy that can be achieved in the crown ether. Thus, the crown ethers in graphene are perfectly preorganized for binding. In the case of transition metal atoms, Ni, Co and Fe atoms are relatively highly bound to 14-crown-4 and develop ferromagnetic graphene as indicated in Fig. 4b . (See Supplementary Fig. 5 ). We expect that these results lead to obvious potential applications in spintronics. In the case of alkaline atoms, we find that the smallest crown ether configurations we examined preferentially bind lithium atoms (see Fig. 4c ). The largest structure we evaluated but have not yet observed, the 18-crown-6 structure, prefers potassium with binding energy of 2.4 eV. This binding energy and that calculated for Na are ~0.4 eV higher than values obtained earlier [33] . Figure 4: Electrostatic potential and selectivity of crown ethers incorporated in graphene. ( a ) Two-dimensional contour plot of electrostatic potential (normalized by maximum value) of 14-crown-4. ( b ) Binding energy of various transition metals in the 14-crown-4 structure in graphene ( c ) Binding energy of alkaline atoms to the 9-crown-1, 10-crown-2, 12-crown-3 and 14-crown-4 structures in graphene. ( d ) Binding energy of alkaline atoms in the 18-crown-6 structure in graphene exceeds that of free 18-crown-6 molecules by about 1.4 eV. Full size image We find that oxygen atoms are incorporated into certain multi-atom vacancies [36] , [37] , namely small holes consisting of even numbers of vacancies. These holes contain five-atom rings (pentagons) after reconstruction as indicated in Fig. 3a–d . This pentagonal site is more reactive than the hexagonal sites because pentagon-induced states are located near the Fermi energy (see Supplementary Fig. 4 ) [37] . As a result, when an oxygen molecule is chemisorbed nearby, for example, at a double vacancy site ( Fig. 3a ), the chemically active pentagonal sites strongly react with the oxygen molecule, pull it apart and then produce a crown ether configuration in the graphene network ( Fig. 3e ). Larger holes containing more five-atom rings (tetra-, hexa- and dodeca vacancies ( Fig. 3b–d )), can be used to produce larger crown ethers in graphene ( Fig. 3e–h ). The experimental images show that these oxygen atoms are incorporated by bridging the dangling bonds of carbon atoms around the perimeter of holes in the graphene lattice. These oxygen–carbon configurations are the simplest form of ether molecules, but in this case, incorporated within the graphene matrix. One can anticipate that the regular arrays of these highly stable crown ether configurations in graphene can be produced by first forming holes using electrons, ions or chemical reactions [38] , [39] , [40] , [41] and then incorporating oxygen (or nitrogen or sulfur) at the hole edges. Oxygen and carbon in the ether configuration at graphene or graphene oxide zig-zag sheet edges have been proposed to exist [42] but has not been imaged by electron microscopy. To understand the reason for this, we examined how oxygen binds to the reconstructed zig-zag edge in graphene. First-principles calculations show that the molecular oxygen on a reconstructed zig-zag edge preferred adsorption at an interfacial pentagon site between two heptagons with each atom of O 2 on top of a C atom. The O 2 molecule does not dissociate. If atomic oxygen is present, each oxygen atom would be singly bonded with a C atom at the pentagon site (C–O bond with binding energy of 1.5 eV). Our 60 keV electron beam would easily eject these weakly bound O atoms. Just as is found with the crown ether molecules, we find that the crown ether configurations in graphene also selectively bind various atoms depending on the ring size. Furthermore, we find the crown ether structure incorporated in graphene generates a much larger binding energy (~1.4 eV) than those obtained with free crown molecules (see Fig. 4d ). The ether-lined cavities in graphene provide the ideal crown ether conformation because of this rigid and planar array of ether dipoles. In summary, we directly observe for the first time that residual oxygen atoms in oxidized graphene form highly stable crown ether configurations within the two-dimensional graphene layer. Density functional calculations show that these oxygen atoms have binding energies of ~9 eV. The calculations indicate that the crown ether configurations in graphene should exhibit selectivity for different cations depending on the crown ether ring size, a key property of individual crown ether molecules, but have the added property of being rigid and planar, prized features sought in preorganized receptors for selective ion binding. The demonstration of ideal crown ethers in graphene with greatly increased binding energy is expected to open up new applications in a wide range of fields, including sensing, analytical separations, nuclear-waste cleanup, hydrometallurgy, biotechnology, catalysis, medicine and information storage. Sample synthesis Suspended specimens of graphene oxide were synthesized by a colloidal chemistry method based on oxidation and exfoliation of graphite. A modified Hummers method [43] was used to oxidize the graphite powders that involves two stages of oxidation, using first K 2 S 2 O 8 and P 2 O 5 in (H 2 SO 4 ), and later a strongly oxidizing mixture (H 2 SO 4 and KMnO 4 ) for total oxidation. Details of the synthesis procedure and additional information on properties can be found elsewhere [44] . STEM–EELS experiments For the STEM study, graphene oxide flakes were deposited on standard holey-carbon-film-covered copper grids and heated several hours at 160 °C in vacuum before loading into the microscope. STEM imaging was performed using a fifth-order aberration-corrected STEM (Nion-UltraSTEM100) with a cold field emission electron source. The microscope was operated at a low accelerating voltage of 60 kV to prevent knock-on damage to the sp 2 bonded carbon in graphene [45] , [46] , [47] . The achievable spatial resolution is ~1.2 Å. The angular range of the collected electrons in medium-angle ADF mode is 58–200 mrad semiangle. EEL spectra were collected using a Gatan Enfina spectrometer with a collection semiangle of 48 mrad. The energy resolution of the EEL spectrum measured from the zero loss full width at half-maximum was 0.3 eV. First-principles calculations First-principles calculations, based on density functional theory, were performed using the Vienna Ab initio Simulation Package. The projector-augmented wave method was used to mimic the ionic cores, while the spin polarized generalized gradient approximation in the Perdew–Burke–Ernzerhof parameterization was employed for the exchange and correlation functional. Atomic positions as well as lattice parameters were optimized using a conjugate gradient algorithm. Ionic and electronic relaxations were performed by applying a convergence criterion of 5 × 10 −2 eV/Å per ion and 10 −4 eV per electronic step, respectively. To calculate the binding energy of oxygen and explore the electronic properties, crown ethers are incorporated into a rectangular region of graphene containing 96 C atoms. The distance between graphene sheets in neighbouring supercells was set to 20 Å to avoid spurious interactions. A k-point sampling of 4 × 4 × 1 was used for the atomic relaxation. How to cite this article : Guo, J. et al. Crown ethers in graphene. Nat. Commun. 5:5389 doi: 10.1038/ncomms6389 (2014).